Cryo-electron tomography reveals ciliary defects underlying humanRSPH1primary ciliary dyskinesia Cilia play essential roles in normal human development and health; cilia dysfunction results in diseases such as primary ciliary dyskinesia (PCD). Despite their importance, the native structure of human cilia is unknown, and structural defects in the cilia of patients are often undetectable or remain elusive because of heterogeneity. Here we develop an approach that enables visualization of human (patient) cilia at high-resolution using cryo-electron tomography of samples obtained noninvasively by nasal scrape biopsy. We present the native 3D structures of normal and PCD-causing RSPH1- mutant human respiratory cilia in unprecedented detail; this allows comparisons of cilia structure across evolutionarily distant species and reveals the previously unknown primary defect and the heterogeneous secondary defects in RSPH1 -mutant cilia. Our data provide evidence for structural and functional heterogeneity in radial spokes, suggest a mechanism for the milder RSPH1 PCD phenotype and demonstrate that cryo-electron tomography can be applied to human disease by directly imaging patient samples. Motile cilia and flagella are highly conserved and ubiquitous organelles that play important roles in propelling cells or liquids along tissues and are critical for the proper function of many human organs and systems [1] , [2] . Primary ciliary dyskinesia (PCD) is a genetically heterogeneous, autosomal recessive, life-shortening disease with a prevalence of ~1/20,000 live births [3] . It is caused by mutations in genes that participate in the biogenesis, assembly and/or function of motile cilia, which manifest in multiple clinical phenotypes, including respiratory distress in term neonates, chronic oto-sino-pulmonary disease, and—in ~50% of patients—organ laterality defects [3] , [4] , [5] , [6] . Diagnosing PCD has traditionally depended on the detection of ultrastructural defects in motile cilia by conventional electron microscopy (EM) [7] . However, about one-third of PCD patients have normal-appearing ciliary ultrastructures by conventional EM [6] —even in cases with known mutations in ciliary proteins [8] . In conventional EM, samples are chemically fixed, heavy-metal-stained, dehydrated and resin-embedded before imaging, which can lead to reduced structure preservation, artefacts and insufficient resolution [9] , [10] . Therefore, advances in imaging techniques are critical for improving our understanding of human cilia and the structural defects that underlie PCD and other ciliopathies. Such techniques would provide new insights into genotype–phenotype and structure–function relationships, and improve diagnostics. Rapid freezing preserves molecular structures in a pristine, fully hydrated state without chemical fixation or staining. For cryo-electron tomography (cryo-ET) of cryo-immobilized samples, ~100 cryo-EM images are recorded at different angles and used to reconstruct the three-dimensional (3D) structure of small intact cells, organelles and macromolecules [9] . Combining cryo-ET with subtomogram averaging is currently the only technique that provides 3D views of native cellular structures, including cilia, with a resolution up to ~3 nm [11] . However, because of the challenges involved in obtaining and preparing sufficient human samples with pristine ultrastructural preservation, cryo-ET has so far not been applied to study human cilia or specimens from human patients in general. Motile cilia share a highly conserved core structure, the axoneme, that is composed of nine outer doublet microtubules (DMTs) surrounding the two central singlet microtubules of the central pair complex (CPC). Radial spokes (RSs) extend from the DMTs and interact with the CPC [11] , [12] . Recently, mutations in the human radial spoke head 1 homologue ( RSPH1 ) gene were shown to cause PCD with a mild disease phenotype characterized by a delayed onset of pulmonary symptoms and the maintenance of better lung function when compared with PCD patients carrying mutations in other genes [13] . Surprisingly, conventional EM studies of human cilia from PCD patients with mutations in RSPH1 or other proposed RS head proteins, RSPH4A and RSPH9, have failed to identify clear RS defects, instead reporting that the majority of these PCD cilia (more than 80% in some individuals) exhibited normal axoneme structure, while a smaller fraction of cilia displayed a heterogeneous set of CPC defects [13] , [14] , [15] , [16] , [17] , [18] . Likewise, a recent (conventional) electron tomography study of chemically fixed cilia from a PCD patient with an RSPH4A mutation characterized the same CPC abnormalities in 3D and did not detect RS defects [19] . These observations differ markedly from RS head protein mutants in the model organism Chlamydomonas [20] , [21] , and raise questions about the role of human RSPH1 in ciliary function and its location in cilia, as well as the precise structural defects, disease mechanism and the cause of the attenuated PCD phenotype of patients with RSPH1 mutations. Here we present the native 3D structures of both normal human and RSPH1 -mutant cilia using cryo-ET to directly image cilia from healthy humans and a PCD patient. We explore the evolutionary conservation and diversity in cilia and flagella, and precisely determine both the previously unknown primary, PCD-causing defects and the heterogeneous secondary CPC abnormalities in the ciliary structure of individuals with RSPH1 gene mutation, providing new insights into the disease mechanism. Improved method for preparing human axonemes for cryo-ET Only specimens with pristine structural preservation and a thickness of less than a few hundred nanometres can be effectively imaged by cryo-EM/ET. Therefore, cryo-ET studies have largely been limited to isolated macromolecular complexes, organelles and small bacterial cells, and cannot be applied to most eukaryotic cells or tissues, including typical clinical samples taken from patients. In contrast to conventional EM, ciliated cells obtained, for example, by nasal scrape biopsy cannot be imaged directly by cryo-ET. Instead, the development of an improved workflow and preparation method for human axonemes was critically important for visualizing the native 3D structure of human cilia by cryo-ET. This required both a noninvasive method for obtaining a sufficient sample of human respiratory cells and a cilia isolation protocol that preserves the native structure of the axonemes. To achieve this, we combined recent advances in culturing, expanding and re-differentiating primary human respiratory epithelial cells [22] , [23] and tested different modifications of widely used cilia isolation procedures [24] , [25] ( Fig. 1 and Supplementary Fig. 1 ). Specifically, a relatively small quantity of human respiratory epithelial cells was noninvasively obtained by nasal scrape biopsy and expanded through multiple passages in cell culture with irradiated fibroblast feeder cells and Rho kinase inhibitor [22] , [23] . When transferred to an air–liquid interface culture system, these conditionally reprogrammed cells re-differentiated into a ciliated, pseudostratified mucociliary epithelium [26] , [27] . This procedure allowed us to amplify the initially harvested primary respiratory epithelial cells ~50-fold. 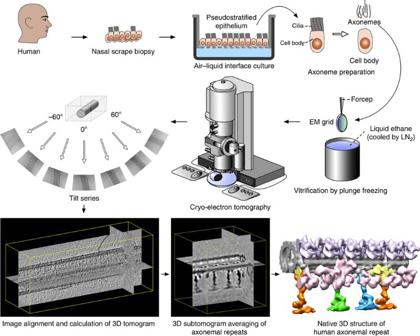Figure 1: Workflow for visualizing the native ultrastructure of human motile cilia. Human respiratory epithelial cells were obtained by nasal scrape biopsy, cultured, expanded and re-differentiated in an air–liquid interface culture. Ciliary axonemes were isolated using our method optimized for cryo-ET. Freshly isolated axonemes were rapidly frozen and transferred to a transmission electron microscope, where tilt series were recorded by stepwise rotation of the axonemes. Image processing was performedin silicoto reconstruct the cryo-tomograms and increase the resolution by subtomogram averaging of the 96-nm repeats. The averaged native 3D structure of the human axonemal repeat can be visualized by isosurface rendering. Figure 1: Workflow for visualizing the native ultrastructure of human motile cilia. Human respiratory epithelial cells were obtained by nasal scrape biopsy, cultured, expanded and re-differentiated in an air–liquid interface culture. Ciliary axonemes were isolated using our method optimized for cryo-ET. Freshly isolated axonemes were rapidly frozen and transferred to a transmission electron microscope, where tilt series were recorded by stepwise rotation of the axonemes. Image processing was performed in silico to reconstruct the cryo-tomograms and increase the resolution by subtomogram averaging of the 96-nm repeats. The averaged native 3D structure of the human axonemal repeat can be visualized by isosurface rendering. Full size image We then tested and optimized methods for cilia isolation from the cultured respiratory epithelial cells. Cryo-ET of cilia isolated by the dibucaine method, which is commonly used to isolate cilia and flagella from protists [20] , [24] , revealed substantial artifactual loss of axonemal components, including dynein arms and one of the CPC microtubules ( Supplementary Fig. 1a–d ). We also tested different modifications of our cilia isolation procedure, which was originally designed for maximal recovery of cilia from cultures of human airway epithelial cells [28] . In the original protocol, cultures of heavily ciliated human respiratory epithelial cells were washed vigorously with a buffer containing calcium and detergent to remove the cilia from the apical cell surface. Although this method is widely used to isolate cilia from epithelial cells [25] , [28] , [29] , we again observed substantial artifactual loss of dynein arms and one of the CPC microtubules in the isolated axonemes ( Supplementary Fig. 1e–h ). Modifications that were successfully tested and incorporated in the final isolation procedure included increasing the concentration of protease inhibitors, pre-incubating the cultures on ice, reducing the speed and duration of the centrifugation steps and minimizing pipetting (see Methods for further details). The most obvious improvement in structural preservation, including for the inner dynein arms (IDAs), was obtained by arresting ciliary motility by incubating the cells on ice before the isolation procedure ( Supplementary Fig. 1i–l ). Although IDAs b and c (based on the labelling system used for Chlamydomonas [30] ) still had weaker electron densities than other IDAs in the axonemal averages ( Supplementary Fig. 1l ), the classification analysis [31] of the averaged axonemal repeats revealed that these IDAs were missing from axonemal repeats that were randomly distributed along the axoneme ( Supplementary Fig. 2a–j ), rather than being a DMT-specific feature such as IDA b (IdaX) in Chlamydomonas flagella [30] , [32] . Randomly missing IDAs could be a common feature of isolated axonemes because we also observed similar effects with IDA extractions for axonemes from other species ( Supplementary Fig. 2k–t ). Our improved preparation method allowed us to visualize the ultrastructure of normal human cilia in unprecedented detail using cryo-ET of rapidly frozen human respiratory ciliary axonemes and subtomogram averaging of the 96-nm axonemal repeats ( Figs 1 , 2 , 3 ; Supplementary Movie 1 ). 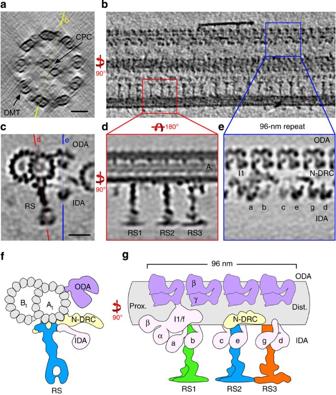Figure 2: Native 3D architecture of normal human ciliary axonemes. (a,b) Tomographic slices show an intact axoneme in cross-sectional (a; 100-nm-thick in proximal-to-distal orientation) and longitudinal (b; 15-nm-thick with proximal on left) views (orientations are consistent in all subsequent figures). Nine DMTs surround the CPC; orientation ofbis indicated ina; boxes inbhighlight 96-nm repeats. (c–e) Tomographic slices show the averaged 96-nm repeat from 12 tomograms of axonemes in cross-sectional (c; 5-nm-thick) and longitudinal (d,e; 10-nm-thick) views; orientations of (d,e) are indicated inc. (f,g) Diagrams of a 96-nm repeat of human motile cilia with four ODAs (dyneins β and γ), six single-headed IDAs (dyneinsa–e,g), the double-headed IDA I1/f, the Nexin–Dynein Regulatory Complex (N-DRC) and three RSs (RS1-3); At/Bt, A- and B-tubules. Scale bars: (a,b) 50 nm, (c–e) 25 nm. Figure 2: Native 3D architecture of normal human ciliary axonemes. ( a , b ) Tomographic slices show an intact axoneme in cross-sectional ( a ; 100-nm-thick in proximal-to-distal orientation) and longitudinal ( b ; 15-nm-thick with proximal on left) views (orientations are consistent in all subsequent figures). Nine DMTs surround the CPC; orientation of b is indicated in a ; boxes in b highlight 96-nm repeats. ( c – e ) Tomographic slices show the averaged 96-nm repeat from 12 tomograms of axonemes in cross-sectional ( c ; 5-nm-thick) and longitudinal ( d , e ; 10-nm-thick) views; orientations of ( d , e ) are indicated in c . ( f , g ) Diagrams of a 96-nm repeat of human motile cilia with four ODAs (dyneins β and γ), six single-headed IDAs (dyneins a – e , g ), the double-headed IDA I1/f, the Nexin–Dynein Regulatory Complex (N-DRC) and three RSs (RS1-3); A t /B t , A- and B-tubules. Scale bars: ( a , b ) 50 nm, ( c – e ) 25 nm. 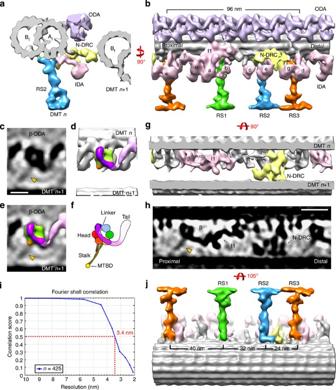Figure 3: Native 3D ultrastructure of the 96-nm axonemal repeat in normal human cilia. (a,b) Isosurface renderings show cross-sectional (a) and longitudinal-front (b) views of the averaged 96-nm repeat from 12 tomograms of axonemes. (c–f) Tomographic slice (c; 1-nm-thick) and isosurface rendering (d) of β-ODA from the averaged 96-nm repeat; note major dynein domains: tail (pink), linker (magenta), head (green) and coiled-coil stalk (arrowheads). A diagram (f) shows the domain organization of dynein, including the microtubule-binding domain (MTBD). (g,h) Isosurface rendering (g) and tomographic slice (h; 1-nm-thick) show the I1 dynein (pink) and N-DRC (yellow); note ultrastructural details, such as the I1 stalk (arrowhead). (i) Resolution of the averaged axonemal repeat (Fourier shell correlation=0.5). (j) Isosurface rendering shows a longitudinal back view of the averaged 96-nm repeat. Scale bars: (c) 10 nm, (h) 20 nm. Full size image Figure 3: Native 3D ultrastructure of the 96-nm axonemal repeat in normal human cilia. ( a , b ) Isosurface renderings show cross-sectional ( a ) and longitudinal-front ( b ) views of the averaged 96-nm repeat from 12 tomograms of axonemes. ( c – f ) Tomographic slice ( c ; 1-nm-thick) and isosurface rendering ( d ) of β-ODA from the averaged 96-nm repeat; note major dynein domains: tail (pink), linker (magenta), head (green) and coiled-coil stalk (arrowheads). A diagram ( f ) shows the domain organization of dynein, including the microtubule-binding domain (MTBD). ( g , h ) Isosurface rendering ( g ) and tomographic slice ( h ; 1-nm-thick) show the I1 dynein (pink) and N-DRC (yellow); note ultrastructural details, such as the I1 stalk (arrowhead). ( i ) Resolution of the averaged axonemal repeat (Fourier shell correlation=0.5). ( j ) Isosurface rendering shows a longitudinal back view of the averaged 96-nm repeat. Scale bars: ( c ) 10 nm, ( h ) 20 nm. Full size image Native 3D structure of the normal human axoneme Using cryo-ET and subtomogram averaging of normal human ciliary axonemes prepared as described above, we visualized the 3D structures at an improved resolution ( Supplementary Table 1 ) compared with previous studies using conventional EM of chemically fixed samples [7] , [13] , [14] , [15] , [16] , [17] , [18] , [33] . The cryo-tomograms show the characteristic 9+2 arrangement of nine DMTs surrounding two CPC singlet microtubules ( Fig. 2a ). Each DMT is composed of 96-nm-long repeat units with highly regular spacing of axonemal complexes, such as the dyneins and RSs ( Fig. 2b ). The radiation sensitivity of ice-embedded biological specimens demands low-dose imaging conditions, leading to noisy raw cryo-tomograms and limited resolution. Therefore, we aligned and averaged 850 subtomographic volumes ( Supplementary Table 1 ), each containing one 96-nm repeat, which significantly increased the resolution of the 3D axonemal reconstruction and the visibility of structural details ( Figs 2 and 3 ; Supplementary Movie 1 ). The averaged axonemal repeat of normal human motile cilia exhibits a similar overall architecture to that of motile cilia and flagella in other organisms [11] , [12] . Specifically, four identical outer dynein arms (ODAs; each ODA contains two dyneins: β- and γ-ODA according to the nomenclature used for Chlamydomonas [30] , [34] ) and six different single-headed IDAs (dyneins a–e and g) are arranged in two rows on the DMTs ( Figs 2c–g and 3a,b ). The double-headed I1 dynein (dynein f) and the Nexin–Dynein Regulatory Complex are located between the ODAs and IDAs ( Figs 2f,g and 3a,b ). The three full-length RSs form typical triplets with a spacing of 40, 32 and 24 nm between RS3 and RS1, RS1 and RS2, and RS2 and RS3, respectively ( Fig. 3b,j ). At the achieved resolution of 3.4 nm ( Fig. 3i ), small features such as individual dynein domains are clearly visible ( Fig. 3c–f ). The improved preservation and resolution of the axonemal structures allowed us to visualize even the single coiled-coil stalk of I1 dynein (arrowhead in Fig. 3h ), which was not possible in prior cryo-ET studies of cilia and flagella in other organisms [11] . Comparison of the axonemal structure across species To explore the evolutionary conservation and diversity of cilia and flagella, we compared the ultrastructure of axonemes from two protists, the unicellular green algae Chlamydomonas and the heterotrophic ciliate Tetrahymena , and from two metazoans, sea urchins and humans. Overall, the relative positions of axonemal components appear highly conserved in all observed species ( Fig. 4 ), including the complex arrangements of the IDAs ( Fig. 4a,d,g,j ). 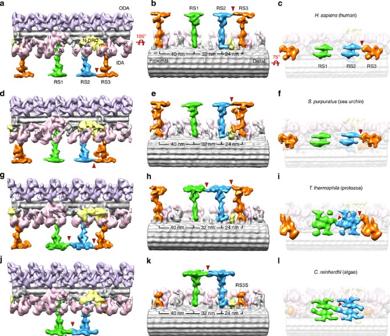Figure 4: Comparison of cilia and flagella across species. (a–l) Isosurface renderings show the averaged 96-nm axonemal repeat from four different species:H. sapiens(a–c; from 12 tomograms),S. purpuratus(d–f; from 9 tomograms),T. thermophila(g–i; from 12 tomograms) andC. reinhardtii(j–l; from 5 tomograms). Each species is shown in three orientations: longitudinal-front (a,d,g,j), back (b,e,h,k) and bottom views (c,f,i,l; looking from the CPC towards the DMT). Red arrowheads highlight the connections between RSs. Figure 4: Comparison of cilia and flagella across species. ( a – l ) Isosurface renderings show the averaged 96-nm axonemal repeat from four different species: H. sapiens ( a – c ; from 12 tomograms), S. purpuratus ( d – f ; from 9 tomograms), T. thermophila ( g – i ; from 12 tomograms) and C. reinhardtii ( j – l ; from 5 tomograms). Each species is shown in three orientations: longitudinal-front ( a , d , g , j ), back ( b , e , h , k ) and bottom views ( c , f , i , l ; looking from the CPC towards the DMT). Red arrowheads highlight the connections between RSs. Full size image The axonemal repeat of human cilia most closely resembles that of sea urchin flagella, whereas it shows greater divergence from Chlamydomonas flagella and Tetrahymena cilia ( Fig. 4 ). For example, each ODA in human and sea urchin axonemes is composed of two dynein heavy chains (human: β and γ; sea urchin: α and β; Fig. 4a,d ), whereas the ODA in the two protists consists of three dynein heavy chains (α, β and γ; Fig. 4g,j ). A similar dichotomy between protists and metazoans is also apparent in the distal half of the RSs with the spoke heads. Although the spacing and architecture of the RS bases appear conserved ( Fig. 4b,e,h,k ), the distal half of the third RS is absent in Chlamydomonas ( Fig. 4k ) and is structurally divergent between the metazoans and Tetrahymena ( Fig. 4c,f,i ). The spoke heads of RS1 and RS2 consist of two structurally identical, rotationally symmetric halves that differ from RS3 in all four species ( Fig. 4c,f,i,l ). However, in the protists, the RS heads of RS1 and RS2 have lateral branches that form a connection between the two heads as well as larger interfaces towards the CPC ( Fig. 4i,l ). In human and sea urchin, the RS1 and RS2 spoke heads resemble a pair of ice skate blades and are clearly separated from each other, whereas the RS2 head connects to the RS3 head ( Fig. 4a–f ); the latter feature is similar to that seen in Tetrahymena ( Fig. 4g–i ). Structural defects in RSPH1 PCD cilia To explore the capability of cryo-ET for studying human disease and to precisely characterize the defects in RSPH1 -mutant cilia, we obtained a nasal scrape biopsy from a PCD patient with compound heterozygous mutations in RSPH1 (subject 1370 (ref. 13 )). As an additional control, we also obtained nasal epithelial cells from the patient’s mother, who was a carrier of one mutation but did not exhibit PCD symptoms. Ciliary axonemes were prepared as described above using our improved procedure and then analysed by cryo-ET in a blinded study. The cryo-tomograms revealed a variety of CPC abnormalities in a subset of RSPH1 -mutant cilia. This was consistent with previous studies of PCD caused by mutations in putative RS head proteins, which revealed a subset of cilia that lacked the CPC (9+0 axoneme) or had one of the nine DMTs translocated to the centre of the axoneme ((8+1)+0) [13] , [14] , [15] , [16] , [17] , [18] , [19] . We found PCD cilia with an apparently normal 9+2 microtubule arrangement ( Fig. 5d ), with one of the CPC microtubules missing (9+1; Fig. 5e ), with the entire CPC missing (9+0; Fig. 5g ), with the CPC replaced by one DMT ((8+1)+0; Fig. 5h ) or with a doubled CPC with four singlet microtubules (9+4; Fig. 5f ). 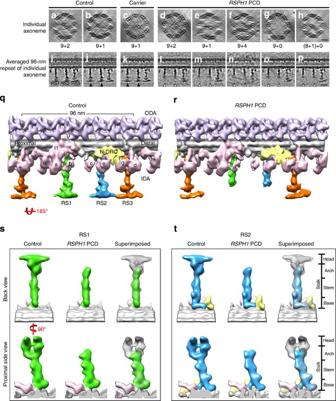Figure 5: Comparison of normal human andRSPH1PCD mutant cilia reveals primary and secondary defects. (a–h) Hundred-nm-thick cross-sectional tomographic slices show individual 3D reconstructed axonemes from normal control (a,b), carrier (c) andRSPH1PCD patient cilia (d–h). (i–p) Ten-nm-thick longitudinal tomographic slices show the averaged 96-nm repeat of individual axonemes from normal control (i,j), carrier (k) andRSPH1PCD patient cilia (l–p). Black and white arrowheads indicate intact and defective RS1/RS2, respectively. (q,r) Isosurface renderings of the averaged 96-nm repeat from normal control (q; 12 tomograms) andRSPH1PCD cilia (r; 20 tomograms). (s,t) Isosurface renderings of the averaged RS1 (s) and RS2 (t) viewed from the longitudinal back (top) and the proximal side (bottom). Differential maps obtained by superimposing the normal control structure (grey) with theRSPH1PCD structure (green or blue) highlight structural defects in mutant cilia; RS domains are indicated (right scales). Scale bars: (a–h) 50 nm, (i–p) 20 nm. Figure 5: Comparison of normal human and RSPH1 PCD mutant cilia reveals primary and secondary defects. ( a – h ) Hundred-nm-thick cross-sectional tomographic slices show individual 3D reconstructed axonemes from normal control ( a , b ), carrier ( c ) and RSPH1 PCD patient cilia ( d – h ). ( i – p ) Ten-nm-thick longitudinal tomographic slices show the averaged 96-nm repeat of individual axonemes from normal control ( i , j ), carrier ( k ) and RSPH1 PCD patient cilia ( l – p ). Black and white arrowheads indicate intact and defective RS1/RS2, respectively. ( q , r ) Isosurface renderings of the averaged 96-nm repeat from normal control ( q ; 12 tomograms) and RSPH1 PCD cilia ( r ; 20 tomograms). ( s , t ) Isosurface renderings of the averaged RS1 ( s ) and RS2 ( t ) viewed from the longitudinal back (top) and the proximal side (bottom). Differential maps obtained by superimposing the normal control structure (grey) with the RSPH1 PCD structure (green or blue) highlight structural defects in mutant cilia; RS domains are indicated (right scales). Scale bars: ( a – h ) 50 nm, ( i – p ) 20 nm. Full size image Subtomogram averaging allowed us to identify additional small structural differences between samples that are not routinely detectable using conventional EM. Intriguingly, our cryo-ET analysis revealed that all cilia from the patient with RSPH1 mutations, including those with an apparently normal 9+2 axonemal arrangement ( Fig. 5d ), showed the same defect in two of the three RSs ( Fig. 5l–p , white arrowheads). Specifically, the head-containing distal regions of RS1 and RS2 were consistently missing in all studied PCD ciliary axonemes from the patient, whereas RS3 appeared normal. These RS defects were not observed in either the normal control sample ( Fig. 5i,j ) or the sample from the heterozygote carrier without PCD symptoms ( Fig. 5k ). Because all averages of individual PCD axonemes revealed a pervasive, homogeneous structural defect ( Fig. 5l–p ), we combined the repeats from multiple PCD axonemes to increase the resolution of the 3D average ( Supplementary Fig. 3c ). Similarly, we calculated total averages from both control groups ( Supplementary Fig. 3a,b ). The absence of the distal regions of RS1 and RS2 is unequivocal in the final PCD average ( Supplementary Fig. 3c , white arrowheads). The head of RS3 also appears slightly weaker than in the controls (compare Supplementary Fig. 3a–c ). A classification analysis focused on RS3 indicates that the weaker electron density is due to the loss of the distal half of RS3 in a fraction (30%) of the PCD axonemal repeats ( Supplementary Fig. 3e,f ); the repeats lacking the RS3 head were randomly distributed among the studied axonemes ( Supplementary Fig. 3d ). Considering the usually observed connection between the heads of RS2 and RS3 in normal human cilia ( Fig. 4a–c , red arrowheads), the absence of RS3 heads in a minority of axonemal repeats of PCD cilia suggests that the RS2 head plays a role in the stable assembly of the RS3 head. We also confirmed that in (8+1)+0 PCD cilia ( Fig. 5h ), the centrally located structure is indeed a DMT and not a modified CPC structure, as indicated by the presence of both (defective) RSs and dyneins in the averaged structure ( Supplementary Fig. 3g–i ). The isosurface renderings of the axonemal averages clearly show that the defects in the 96-nm repeat of RSPH1 -mutant human cilia are specific to the distal regions of RS1 and RS2, whereas all other DMT-associated structures appear normal (compare Fig. 5q,r ). Both RS1 and RS2 of RSPH1 PCD cilia display the same defects, that is, the entire spoke head and part of the following arch region are missing ( Fig. 5r–t ; Supplementary Movie 2 ); the rest of the stalk and base structures of RS1 and RS2 appear to be identical between normal controls and RSPH1 -mutant cilia. Because these structural defects are pervasive in all RSPH1 -mutant cilia and are consistent with the fact that RSPH1 encodes an RS protein homologue, they represent the primary defects in RSPH1 PCD cilia, while the heterogeneous abnormalities seen in the CPC are secondary defects. Until the present study, cryo-ET was not used to study human clinical samples mainly because of challenges surrounding the collection and preparation of sufficient quantities of human samples with good structural preservation. Here, we successfully combined recent improvements in the culture and expansion of respiratory epithelial cells [22] , [23] and developed an isolation procedure for human ciliary axonemes that is optimized for structure preservation and is compatible with high-resolution cryo-ET imaging ( Fig. 1 ). These improvements allowed us to use cryo-ET and subtomogram averaging to determine the native 3D structures of human cilia with 3- to 4-nm resolution, which is sufficient for observing features as small as the coiled-coil stalks of dynein motors ( Fig. 3c–h ). Moreover, the application of recently established classification methods [31] can efficiently detect and localize heterogeneities and therefore allowed us to recognize the normal variability that is typically present in clinical samples ( Supplementary Figs 2,3d–f ) and distinguish it from pervasive disease-specific defects. Using only pristine axonemal repeats, our averaged structure represents the 3D molecular architecture of normal human motile cilia in their native state ( Fig. 3 ). Although the overall structures of cilia and flagella are highly conserved, the structural diversity observed across species both in the present study and in previous studies warrants caution in generalizing findings from model organisms such as Chlamydomonas to understand human ciliary function and the defects and mechanisms underlying human ciliopathies. In all species examined with three RSs per axonemal repeat, RS3 is structurally distinct from RS1 and RS2 ( Fig. 4 ), suggesting a potentially unique proteome for RS3. This is strongly supported by our observation that mutations in RSPH1 only affect the structures of RS1 and RS2 but not RS3 ( Fig. 5 ). Twenty-three proteins are currently known to constitute RS1 and RS2 in Chlamydomonas [20] , [35] , [36] . However, little is known about either the proteome or the function of RS3 because knowledge of RSs is mainly derived from Chlamydomonas , which lacks a major portion of RS3. In Chlamydomonas , the absence of the RS1 and RS2 heads results in complete flagellar paralysis [20] , [21] , [37] , whereas similar defects in RS1 and RS2 cause only a moderate motility defect in human RSPH1 -mutant cilia [13] , suggesting an important role for intact RS3 in ciliary motility. Future studies are required to determine the RS3 proteome, its specific function in motility and why RS3 is present in humans and other organisms but is reduced in Chlamydomonas . The presence of secondary defects in the RSPH1 -mutant PCD cilia ( Fig. 5f–h ) suggests that both intact RSs and RS–CPC interactions are critical for proper and stable CPC assembly. When the RSs are not intact, the increased physical space in the centre of the axonemal cylinder could lead to the presence of an additional CPC ( Fig. 5f ) or to CPC destabilization, which raises interesting questions about the templating and assembly mechanism of the CPC. Similar CPC defects were also observed in the Chlamydomonas pf14 mutant, which lacks RS1 and RS2 (ref. 38 ). Our analysis has precisely determined both the primary and the secondary defects in RSPH1- mutant PCD cilia ( Figs 5 and 6 ). Relating these structural defects to their motility phenotypes and to PCD clinical symptoms provides a deeper understanding of the structure–function relationships of the axonemal machinery in human cilia and the PCD disease mechanism. In particular, we recently reported that patients with mutations in RSPH1 have a delay in early clinical manifestations of the disease and a ‘milder’ lung disease [13] . RSPH1 patients have a lower incidence of neonatal respiratory distress, and they maintain better lung function compared with PCD individuals with mutations in other genes [13] . In our cultured samples, the vast majority of cilia beat with near-normal frequencies but exhibited abnormal circular patterns [13] . This circular motility may provide a low but substantial rate of mucociliary clearance, resulting in a less severe PCD phenotype in RSPH1 patients compared with those observed in individuals with other PCD mutations. Recently published data from a murine model suggest that maintaining as little as 20% of the normal mucociliary clearance rate can greatly reduce the severity of PCD [39] . Therefore, our data suggest that the remaining intact RS3 provides sufficient ciliary function to result in the milder disease phenotype in RSPH1 PCD patients, making RS3 a potential target for therapeutic interventions in ciliopathy patients (for example, improve the motility of RSPH1 PCD cilia by upregulating the function of RS3). 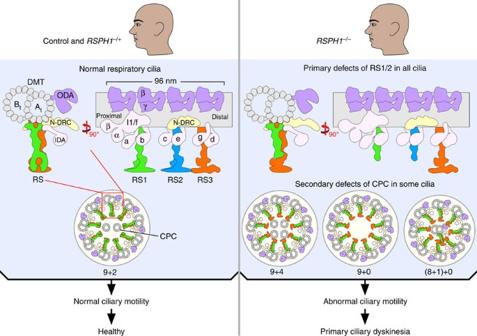Figure 6: Cryo-ET provides new insights into the structural basis of humanRSPH1PCD. Schematic representation of the comparison between the native 3D structures of respiratory cilia from normal controls (includingRSPH1−/+carrier) and PCD patient (RSPH1−/−). Our cryo-ET analysis revealed both unprecedented structural details of normal respiratory cilia (left column) and the previously unknown, yet consistently present primary RS defects and the heterogeneous secondary CPC defects in theRSPH1-mutant cilia (right column). At/Bt, A- and B tubules. Figure 6: Cryo-ET provides new insights into the structural basis of human RSPH1 PCD. Schematic representation of the comparison between the native 3D structures of respiratory cilia from normal controls (including RSPH1 −/+ carrier) and PCD patient ( RSPH1 −/− ). Our cryo-ET analysis revealed both unprecedented structural details of normal respiratory cilia (left column) and the previously unknown, yet consistently present primary RS defects and the heterogeneous secondary CPC defects in the RSPH1 -mutant cilia (right column). A t /B t , A- and B tubules. Full size image In conclusion, our proof-of-concept translational study demonstrates that state-of-the-art cryo-ET imaging of patient samples can provide unique insights into human disease. We introduced an improved protocol that makes it feasible to perform cryo-ET of human cilia, including those of ciliopathy patients, and provided the native 3D structure of normal human motile cilia as a reference, which will greatly increase the resolution and reliability of future ultrastructural studies. We identified the previously undetected primary RS1 and RS2 defects in cilia from an RSPH1 PCD patient, whereas RS3 was intact. These data are consistent with the predicted homology of RSPH1 to RS head proteins, clarify previously puzzling observations obtained by conventional EM, which could only resolve the secondary CPC abnormalities and offer an explanation for why this particular variant of PCD has a clinically attenuated phenotype. Culture of human airway and nasal epithelial cells Control human airway epithelial cell cultures of non-PCD, non-cystic fibrosis cells were used to determine the normal structure of human motile cilia. Human airway epithelial cells were obtained from the UNC Cell and Tissue Culture Core Facility under protocols approved by the Institutional Review Board for the Protection of the Rights of Human subjects at UNC. All human tissues were obtained with informed consent. Cells were cultured at an air–liquid interface on collagen-coated culture inserts (Millicell, Millipore) until they were heavily ciliated [40] . Briefly, 10 6 human airway epithelial cells were plated on 4.2-cm 2 Millicell cell culture inserts (Millipore) coated with 250-μg human type IV collagen (Sigma). An air–liquid interface was established when the cells were confluent (~3 days) by removing the apical media and feeding from the basolateral side. Cultures were fed 3 × weekly with a 50:50 mixture of LHC-basal and DMEM-H media supplemented as described (ALI media [40] ) for 2 weeks, after which cultures were fed 2 × weekly. The apical surface of the cultures was washed with PBS to remove mucus and cell debris along with each media change. Ciliated-cell differentiation was monitored by phase contrast microscopy and cultures became heavily ciliated after ~4 weeks at the air–liquid interface. Nasal epithelial cells from a PCD patient with two mutations in the RSPH1 gene and a heterozygous parent (carrier) were obtained by nasal scrape biopsy under protocols approved by the Institutional Review Board for the Protection of the Rights of Human subjects at UNC [13] . Cells were first expanded on plastic dishes in media containing fibroblast-conditioned media and Rho kinase inhibitor, Y-27632 (ref. 23 ). After expansion, the cells were passaged on collagen-coated Millicells and cultured at an air–liquid interface as described above until ciliated-cell differentiation occurred. Isolation of human ciliary axonemes Ciliary axonemes were isolated from human airway and nasal epithelial cell cultures using a modified version of a previously published method [28] . The final procedure was as follows: first, the apical surfaces of well-differentiated cultures were gently washed twice for 5 min with PBS to remove mucus and cell debris. Then, the medium was removed, the apical and basal compartments of the air–liquid interface culture dish were filled with ice-cold PBS and the culture dish was placed on a bed of ice for ~5 min, at which time ciliary activity was reduced to near zero. The PBS solution was removed and ice-cold deciliation buffer (10 mM Tris pH 7.5, 50 mM NaCl, 10 mM CaCl 2 , 1 mM EDTA, 0.1% Triton X-100, 7 mM β-mercaptoethanol, 1% protease inhibitor cocktail (Sigma P8340)) was gently added to the apical surface of the culture (50 μl per 12-mm insert). The culture was incubated for 2 min (without shaking, different from previous protocols), and then the apical solution, which contained the cilia, was removed and transferred to a microcentrifuge tube. Mucus and cellular debris were gently pelleted by centrifugation at 4 °C for 1 min at 500 × g . The supernatant was again centrifuged at 4 °C for 5 min at 5,000 × g to collect the ciliary axonemes. The axonemal pellet was gently dispersed in resuspension buffer (30 mM HEPES pH 7.3, 1 mM EGTA, 5 mM MgSO 4 , 0.1 mM EDTA, 25 mM NaCl, 1 mM dithiothreitol, 1% protease inhibitor cocktail and 100 g ml −1 soybean trypsin inhibitor (Sigma T9128)) and kept on ice until cryo-sample preparation. Ciliary samples from the heterozygous control (carrier) and the PCD patient were analysed by cryo-ET with the investigator blinded to the identity of the samples. Flagella and cilia preparation from model organisms Live sea urchin sperms were collected from adult male Strongylocentrotus purpuratus (purchased from Monterey Abalone Co. (Monterey, CA)) after inducing the spawning by the injection of 1–2 ml of 0.5 M KCl into the perivisceral cavity of sea urchins [41] , [42] . The sperms were diluted in artificial seawater (360 mM NaCl, 50 mM MgCl 2 , 10 mM CaCl 2 , 10 mM KCl and 30 mM HEPES, pH 8.0) with the ATPase inhibitor erythro-9-[3-(2-hydroxynonyl)]-adenine (2 mM) [43] . After a 5-min incubation at ~16 °C, the sample was viewed under a light microscope to confirm that the sperms were completely immotile. Tetrahymena axonemes were isolated form T. thermophila (strain CU428) cells. Cells were grown to a density of ~3 × 10 5 ml −1 and collected by centrifugation at 3,000 × g , washed with 10 mM Tris pH 7.5, centrifuged at 1,500 × g and resuspended in 10 mM Tris pH 7.5, 50 mM sucrose, 10 mM CaCl 2 with protease inhibitors. Cilia were detached from the cells by the pH-shock method [44] and purified by two centrifugation steps at 1,860 × g for 5 min each. Purified cilia were collected by centrifugation at 10,000 × g for 15 min and demembranated in HMEEK buffer (30 mM HEPES, pH 7.4, 25 mM KCl, 5 mM MgSO 4 , 0.1 mM EDTA and 1.0 mM EGTA) with 1% IGEPAL CA-630 (Sigma-Aldrich, St Louis, MO) for 20 min. The axonemes were then collected by centrifugation at 10,000 × g for 10 min and resuspended in HMEEK buffer without IGEPAL CA-630. C. reinhardtii axonemes were isolated from a pseudo-wild-type strain (pf2-4::PF2-GFP (green fluorescent protein)) [45] . This strain is a rescued mutant that was obtained by transforming the nexin–dynein regulatory complex-defective pf2 -mutant strain with a GFP-tagged wild-type PF2 gene [45] , [46] . This strain is biochemically, structurally and phenotypically indistinguishable from the wild type [45] . Cells growing in liquid Tris-acetate-phosphate medium were harvested, washed and resuspended in pH-shock buffer containing 10 mM HEPES, pH 7.4, 1 mM SrCl 2 , 4% sucrose and 1 mM dithiothreitol. Flagella were detached from the cells using the pH-shock method [44] . Then, the solution was supplemented with 5 mM MgSO 4 , 1 mM EGTA, 0.1 mM EDTA and 100 μg ml −1 aprotinin, pepstatin and leupeptin, and centrifuged at 1,800 × g for 10 min at 4 °C. The supernatant containing the flagella was collected and purification of the flagella was conducted by two centrifugation steps at 2,400 × g for 10 min at 4 °C with a 20% sucrose cushion. Purified flagella were demembranated with 0.1% IGEPAL CA-630 (Sigma-Aldrich) and axonemes were collected by centrifugation at 35,000 × g for 1 h at 4 °C. The axoneme pellet was washed with HMEEN buffer (30 mM HEPES, pH 7.4, 5 mM MgSO 4 , 1 mM EGTA, 0.1 mM EDTA, 25 mM NaCl and 0.1 μg ml −1 aprotinin, leupeptin and pepstatin) and then resuspended in HMEEN buffer for cryo-sample preparation. Cryo-sample preparation and cryo-electron tomography Isolated axoneme samples (3 μl) and a fivefold-concentrated 10-nm colloidal gold solution (1 μl, Sigma-Aldrich) were applied to glow-discharged Quantifoil holey carbon grids (R2/2, Quantifoil Micro Tools GmbH, Germany), which were loaded on a homemade plunge freezing device. The grid was blotted with filter paper for 1.5–2.5 s and immediately frozen by plunging into liquid ethane cooled by liquid nitrogen. The vitrified samples were then stored in liquid nitrogen until examined by cryo-ET. Single axis tilt series were acquired using a Tecnai F30 transmission electron microscope (FEI, Hillsboro, OR), operated at 300 keV and equipped with a field emission gun and a post-column energy filter (Gatan, Pleasanton, CA). Cryo-samples were transferred into the microscope with a cryo-holder (Gatan) and kept at ~170 °C. The samples were imaged under low-dose conditions in zero-loss mode (20 eV slit width) with −6 or −8 μm defocus. Flagella and axonemes that seemed well preserved and not (or only slightly) compressed by EM inspection were selected for electron tomography. Tilt series of images were collected by stepwise rotation of the sample from −65 to +65° at 1.5–2.5° increments using the SerialEM software [47] . The cumulative electron dose was limited to ~100 e Å −2 for individual tilt series to avoid radiation damage. All images were recorded on a 2 × 2 k charge-coupled device camera (Gatan) at a nominal magnification of × 13,500. The pixel size was ~1 nm. Image processing The tilt series images with sufficient gold fiducial markers for alignment were aligned and reconstructed into 3D tomograms using the IMOD software with weighted backprojection [48] . Tomograms of compressed flagella or axonemes (caused by embedding in too thin ice during cryo-sample preparation) were excluded from further subtomogram averaging and analysis. Subtomogram averaging with missing wedge compensation was performed with the PEET software [49] to achieve enhanced signal-to-noise ratio and improved resolution. Two different aligning strategies were employed: (a) to optimize the alignment accuracy for the entire 96-nm axonemal repeat, subtomograms containing the 96-nm axonemal repeats were extracted from the tomograms, aligned and averaged in 3D ( Figs 2 , 3 , 4a,b,d,e,g,h,j,k and 5a–r and Supplementary Figs 1–3 ); (b) to resolve the RSs at the highest possible detail, smaller subtomograms containing the structures of interest were extracted, locally aligned (calculated centred on the structure of interest) and averaged ( Figs 4c,f,i,l and 5s,t ). The resulting averages of each RS with local alignment provide a slightly higher level of detail. To analyse the heterogeneity of the axonemal structures, we further performed automated classification on the subtomograms using a clustering approach implemented into the PEET programme [31] . The classified 3D volume was limited to the structures of interest using appropriate masking. The resolution of the resulting averages was estimated in a 20-nm 3 subvolume in the centre of 96-nm axonemal repeat using the Fourier shell correlation method and the 0.5 criterion [50] . The IMOD software [42] and the UCSF Chimera package [51] were used for visualization of the tomographic slices and 3D visualization by isosurface rendering, respectively. How to cite this article: Lin, J. et al. Cryo-electron tomography reveals ciliary defects underlying human RSPH1 primary ciliary dyskinesia. Nat. Commun. 5:5727 doi: 10.1038/ncomms6727 (2014). Accession codes: The cryo-ET map of the human 96-nm axonemal repeat from a normal human control has been deposited in the EM Data Bank under accession code EMD- 5950 .